Targeted drug delivery using genetically engineered diatom biosilica The ability to selectively kill cancerous cell populations while leaving healthy cells unaffected is a key goal in anticancer therapeutics. The use of nanoporous silica-based materials as drug-delivery vehicles has recently proven successful, yet production of these materials requires costly and toxic chemicals. Here we use diatom microalgae-derived nanoporous biosilica to deliver chemotherapeutic drugs to cancer cells. The diatom Thalassiosira pseudonana is genetically engineered to display an IgG-binding domain of protein G on the biosilica surface, enabling attachment of cell-targeting antibodies. Neuroblastoma and B-lymphoma cells are selectively targeted and killed by biosilica displaying specific antibodies sorbed with drug-loaded nanoparticles. Treatment with the same biosilica leads to tumour growth regression in a subcutaneous mouse xenograft model of neuroblastoma. These data indicate that genetically engineered biosilica frustules may be used as versatile ‘backpacks’ for the targeted delivery of poorly water-soluble anticancer drugs to tumour sites. Research on porous silica-based particles has demonstrated their suitability for drug-delivery applications due to their extended drug release profiles and high efficacy in delivering hydrophobic drugs [1] . Indeed, the application of nanoporous silica materials for drug delivery is a cornerstone of the burgeoning field of nanomedicine [2] . The most intensively investigated silica materials for drug delivery are mesoporous silica and oxidized porous silicon [3] . Both feature high surface area, thermal stability, tunable pore size, chemical inertness, excellent biocompatibility and (at least in the case of porous silicon) biodegradability [4] . A significant drawback for the use of these materials is that their synthesis requires toxic chemicals (in particular silanes and hydrofluoric acid) and is time-consuming and costly. A potential alternative to synthetic mesoporous silica are diatoms, the large and abundant group of single-celled photosynthetic microorganisms, which are encapsulated in biomineralized silica walls also called frustules. The hallmark of diatom biosilica is the hierarchical arrangement of three-dimensional patterns of pores with diameters in the nano- to microscale range (20 nm–2 μm) [5] . Diatom biosilica exhibits both high surface area ( ∼ 100 m 2 g −1 ) [6] and high mechanical stability [7] . Losic and colleagues [8] , [9] have pursued the idea of using diatom biosilica as a biocarrier for applications in oral and implant drug delivery, and have demonstrated their potential to replace synthetic silica-based materials. Chemical functionalization allows for the tailoring of drug binding and release properties [10] , [11] , and for the covalent immobilization of functional antibody molecules to diatom silica [12] , [13] . Combining both antibody attachment and drug loading on the same diatom silica particle should allow for targeted delivery of the drug to specific locations in vivo , for example, to cancer cells. Active targeting of drug-delivery vehicles using antibodies that target tumour cells via cognate cell membrane receptors overexpressed in cancer has been shown to improve therapeutic outcomes in cancer and prevent off-target delivery-related side effects [14] . However, simultaneous binding of drugs and antibodies to diatom silica particles has not been achieved and has hardly been investigated for synthetic mesoporous silica materials [15] . To date, there is only one successful example that has demonstrated the targeted delivery of doxorubicin to tumour-bearing tissue in mice using antibody-functionalized mesoporous silica nanoparticles [16] . In the present study, we have aimed to develop a generic method for the simultaneous attachment of both antibodies and hydrophobic drug molecules to diatom biosilica, without the use of organic solvents and covalent cross-linking. The strategy for this method involves (a) the incorporation of antibody-binding protein domains into the diatom biosilica through genetic engineering and (b) the incorporation of drug molecules into silica-binding carriers. To achieve (a), we use a recently developed method termed live diatom silica immobilization (LiDSI) [17] , [18] , to incorporate GB1, an immunoglobulin G (IgG)-binding domain of protein G [19] , into the biosilica of the diatom T. pseudonana in vivo and investigate the attachment of IgG antibodies to the genetically engineered biosilica. To achieve (b), we use an established method to encapsulate hydrophobic drug molecules into cationic micelles and liposomes [20] , [21] , followed by investigations on their biosilica-binding properties and the release of the drug molecules. This two-step strategy is necessary, as loading of the diatom frustules with a hydrophobic drug from an organic solvent would denature the antibody. This approach leads to multistage drug-delivery vehicles [19] , [20] , where drug-loaded nanoscale vehicles can be deployed once the biosilica has attached to tumour cells ( Fig. 1 ) [20] , [21] . 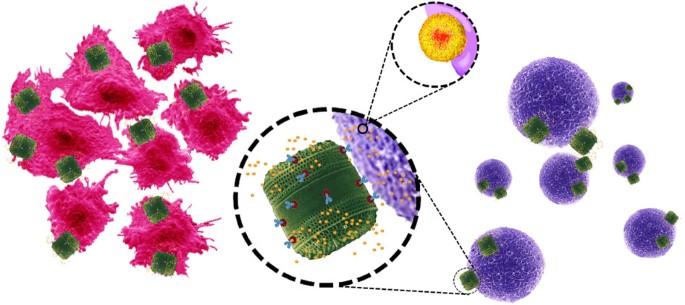Figure 1: The principle of action of the genetically engineered biosilica therapeutic nanoparticles. Genetically engineered diatom biosilica (green) containing liposome-encapsulated drug molecules (yellow) can be targeted to both adherent neuroblastoma cells (red) and lymphocyte cells in suspension (purple) by functionalizing the biosilica surface with cell-specific antibodies. Liposome-encapsulated drug molecules are released from the biosilica carrier in the immediate vicinity of the target cells (inset). Figure 1: The principle of action of the genetically engineered biosilica therapeutic nanoparticles. Genetically engineered diatom biosilica (green) containing liposome-encapsulated drug molecules (yellow) can be targeted to both adherent neuroblastoma cells (red) and lymphocyte cells in suspension (purple) by functionalizing the biosilica surface with cell-specific antibodies. Liposome-encapsulated drug molecules are released from the biosilica carrier in the immediate vicinity of the target cells (inset). Full size image Functional display of GB1 on genetically modified diatoms T. pseudonana ( Fig. 2 ) was chosen as the model diatom for the present study, because a method has been established for the in vivo incorporation of foreign proteins into the biosilica of this diatom, using genetic engineering [17] , [18] . This method, coined LiDSI, is based on introducing a synthetic gene that encodes the protein of interest fused to an amino-terminal signal peptide (S) and the peptide T8 (ref. 18 ) into the diatom’s genome. Both S (17 amino acids) and T8 (37 amino acids) are derived from silaffin-3 (231 amino acids), which is a natural component of T. pseudonana biosilica [22] . The combination of S and T8 acts as intracellular address tag for permanently anchoring proteins into the biosilica during its formation [18] , [23] . Until now, LiDSI has been used only to incorporate green fluorescent protein (GFP) and enzymes into biosilica [17] , [18] , [24] . 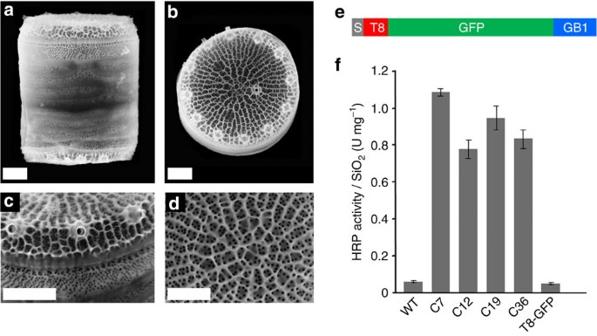Figure 2: SEM images ofT. pseudonanabiosilica and analysis of IgG–HRP binding toT. pseudonanabiosilica. (a) Side view and (b) top view of cylinder-shaped biosilica from a single diatom cell. (c,d) Details of the biosilica structure showing the highly porous surface. (e) Schematic structure of the S–T8–GFP–GB1 fusion protein. S, N-terminal signal peptide of silaffin Sil3 (amino acids 1–17); T8, silica targeting domain from silaffin-3 (amino acids 164–200); GFP, enhanced GFP; GB1, IgG binding domain B1 from protein G. It is noteworthy that the N-terminal signal peptide S becomes removed by the endogenous signal peptidase during intracellular transport of the fusion protein18,23. (f) IgG binding was determined by HRP activity measurements of diatom biosilica after incubation with IgG–HRP and removal of unbound IgG–HRP. SiO2mass of biosilica was determined using the silicomolybdate assay as described18. IgG–HRP binding to biosilica from wild type (WT), from four GFP-fluorescent transformant clones that express the T8–GFP–GB1 fusion protein (C7, C12, C19 and C36) and from a previously described transformant clone that strongly expresses the T8–GFP fusion protein18. Experiments were performed in biological triplicates (n=3). Error bars represent s.d. Scale bars, 1 μm (a–c) and 200 nm (d). Figure 2: SEM images of T. pseudonana biosilica and analysis of IgG–HRP binding to T. pseudonana biosilica. ( a ) Side view and ( b ) top view of cylinder-shaped biosilica from a single diatom cell. ( c , d ) Details of the biosilica structure showing the highly porous surface. ( e ) Schematic structure of the S–T8–GFP–GB1 fusion protein. S, N-terminal signal peptide of silaffin Sil3 (amino acids 1–17); T8, silica targeting domain from silaffin-3 (amino acids 164–200); GFP, enhanced GFP; GB1, IgG binding domain B1 from protein G. It is noteworthy that the N-terminal signal peptide S becomes removed by the endogenous signal peptidase during intracellular transport of the fusion protein [18] , [23] . ( f ) IgG binding was determined by HRP activity measurements of diatom biosilica after incubation with IgG–HRP and removal of unbound IgG–HRP. SiO 2 mass of biosilica was determined using the silicomolybdate assay as described [18] . IgG–HRP binding to biosilica from wild type (WT), from four GFP-fluorescent transformant clones that express the T8–GFP–GB1 fusion protein (C7, C12, C19 and C36) and from a previously described transformant clone that strongly expresses the T8–GFP fusion protein [18] . Experiments were performed in biological triplicates ( n =3). Error bars represent s.d. Scale bars, 1 μm ( a – c ) and 200 nm ( d ). Full size image To incorporate GB1 into T. pseudonana biosilica ( Fig. 2a–d ), the fusion gene S - T8 - GFP - GB1 ( Fig. 2e ) was constructed via recombinant DNA technology and then incorporated into the genome of the diatom T. pseudonana and expressed using established protocols [25] . The GFP tag was introduced to identify transformants that express the GB1 fusion protein, by using fluorescence microscopy. The biosilica from the four transformant clones (C7, C12, C19 and C36) that exhibited the highest fluorescence intensity was tested for IgG binding activity using an IgG-horseradish peroxidase (HRP) conjugate. The biosilica from each of the GFP fluorescent transformants exhibited over tenfold more HRP activity per mass unit of biosilica than the wild-type cells ( Fig. 2f ), indicating that the biosilica from the transformants contained specific IgG-binding protein domains. To investigate whether the T8–GFP region of the fusion proteins contributes to IgG–HRP binding, the assay was repeated with biosilica isolated from a transformant that expressed the fusion protein S–T8–GFP [18] , [23] , which lacks the GB1 domain. The T8–GFP-containing biosilica exhibited <5% IgG–HRP binding relative to the T8–GFP–GB1 containing clone C7 ( Fig. 2f ). Together, the data demonstrate that the GB1 domain is functionally displayed on the biosilica surface of transformants expressing the T8–GFP–GB1 fusion protein [23] . As the biosilica from clone C7 exhibited the highest IgG-binding capacity, it was used for all further experiments in this study. To directly visualize the IgG binding to diatom biosilica and thus confirm its specificity, several IgGs conjugated to DyLight 549 (a red fluorescent molecule) were incubated with T8–GFP–GB1–biosilica (GB1–biosilica) and subsequently analysed by fluorescence microscopy. T8–GFP–biosilica was used as a negative control. As expected, DyLight549-conjugated IgGs bound to GB1-bearing biosilica but not to negative control biosilica, which exhibited GFP fluorescence only ( Fig. 3 ). Quantitative analysis revealed that >99% of the GB1–biosilica frustules bound DyLight549-conjugated IgG, as revealed by the yellow colour of the merged fluorescence images. By contrast, no yellow biosilica frustules were observed for the control sample. These results confirm that GB1–biosilica specifically binds to IgG. 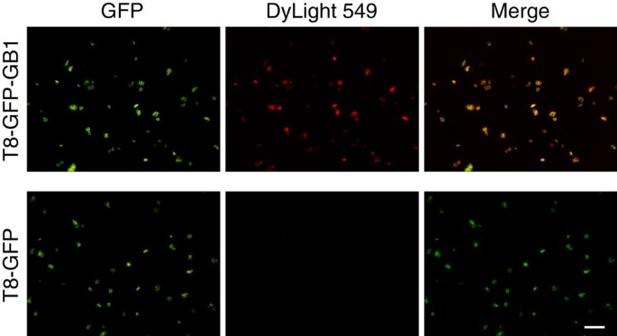Figure 3: Epifluorescence microscopy analysis of binding of DyLight549-conjugated IgG to GFP-fluorescentT. pseudonanabiosilica. T8–GFP–GB1–biosilica- and T8–GFP-bearing biosilica (control) were incubated with DyLight549-conjugated mouse antihuman IgG (n=3). Fluorescence images from the same area of view were recorded separately using different filter sets for the green chromophore (‘GFP’) and the red chromophore (‘DyLight549’). Yellow colour in the overlay of the red and green fluorescence channels (‘Merge’) indicates binding of IgG to the biosilica. Scale bar, 20 μm. Figure 3: Epifluorescence microscopy analysis of binding of DyLight549-conjugated IgG to GFP-fluorescent T. pseudonana biosilica. T8–GFP–GB1–biosilica- and T8–GFP-bearing biosilica (control) were incubated with DyLight549-conjugated mouse antihuman IgG ( n =3). Fluorescence images from the same area of view were recorded separately using different filter sets for the green chromophore (‘GFP’) and the red chromophore (‘DyLight549’). Yellow colour in the overlay of the red and green fluorescence channels (‘Merge’) indicates binding of IgG to the biosilica. Scale bar, 20 μm. Full size image Next, we estimated the density of bound IgG molecules by scanning electron microscopy (SEM) imaging, with anti-rat IgG antibody conjugated to 10 nm gold nanoparticles at various positions along the biosilica. The SEM images presented in Supplementary Fig. 1 show the gold nanoparticles as 10 nm white dots distributed along the surface of the biosilica. The presence of the gold nanoparticles was confirmed by energy-dispersive X-ray analysis (EDAX). From the SEM images, the density of IgG-binding sites on GB1–biosilica was determined to be 35±4 (mean±s.e.m.) μm −2 . Having characterized the IgG-binding specificity and capacity of GB1–biosilica, we then investigated its function in biological systems. Cell targeting with antibody-labelled diatom biosilica We first investigated whether antibody-labelled GB1–biosilica can specifically bind to surface-attached cells that display the corresponding antigen. Microarrays of HR1K Burkitt’s lymphoma cells (B cells) and Jurkat cells (T cells) were generated by capturing the cells on microarray surfaces that display spots of immobilized anti-CD45 antibody ( Supplementary Fig. 2 ) [26] , [27] , [28] . It is noteworthy that both cell types express the antigen CD45. GB1–biosilica was labelled with rituximab; this antibody is specific for the antigen CD20, which is present only on B cells. The captured cell microarrays were incubated with this anti-CD20-labelled GB1–biosilica and, after extensive washing, were analysed by epifluorescence microscopy. The majority of B cells (54% of 503 cells) were associated with diatom biosilica frustules ( Fig. 4a ), whereas not a single T cell showed attached biosilica frustules (0% of 494 cells; Fig. 4b ). In an additional control experiment, the cell microarrays were exposed to T8–GFP–biosilica (which lacks the GB1 domain) that had been pre-incubated with anti-CD20 antibody. As expected, no attachment of biosilica frustules to B cells was observed ( Supplementary Fig. 3 ). These results confirm that the GB1 domain is necessary for labelling the diatom biosilica with antibodies that target cell surfaces. 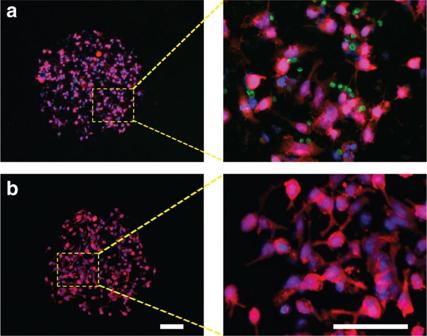Figure 4: Interaction of anti-CD20 antibody-labelled GB1–biosilica with B and T cells captured on an anti-CD45 antibody microarray. The left panels show epifluorescence microscopy images of cells captured on microarray spots after incubation with anti-CD20 antibody-labelled biosilica (n=3). The right panels show higher magnification images within the spots. Green: biosilica (GFP-labelled), red: actin (TRITC-labelled phalloidin), blue: nucleus (Hoechst 33342). (a) B cells (Burkitt’s lymphoma HR1K cells) and (b) T cells (Jurkat cells). Scale bars, 100 μm (all). Figure 4: Interaction of anti-CD20 antibody-labelled GB1–biosilica with B and T cells captured on an anti-CD45 antibody microarray. The left panels show epifluorescence microscopy images of cells captured on microarray spots after incubation with anti-CD20 antibody-labelled biosilica ( n =3). The right panels show higher magnification images within the spots. Green: biosilica (GFP-labelled), red: actin (TRITC-labelled phalloidin), blue: nucleus (Hoechst 33342). ( a ) B cells (Burkitt’s lymphoma HR1K cells) and ( b ) T cells (Jurkat cells). Scale bars, 100 μm (all). Full size image We then investigated whether antibody-labelled biosilica can also bind to cells in suspension. Anti-CD20 antibody-labelled GB1–biosilica was incubated with B and T cells stained with CellTracker Orange. Using fluorescence microscopy, the antibody-labelled GB1–biosilica was frequently observed surrounding B cells ( Fig. 5a ), whereas the same biosilica frustules were unable to attach to T cells ( Fig. 5b ). The same result was obtained when 1:1 mixtures of B cells (stained with CellTracker Orange) and T cells (stained with CellTracker Blue) were incubated with anti-CD20 antibody-labelled GB1–biosilica ( Fig. 5c ). This result demonstrates that GB1–biosilica frustules labelled with the anti-CD20 antibody can specifically target B cells under conditions that approximate the B-cell to T-cell ratio in human blood. 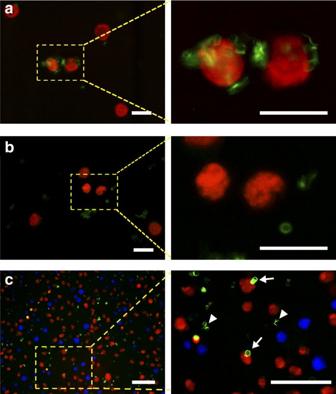Figure 5: Interaction of anti-CD20 antibody-labelled GB1–biosilica with B and T cells in suspension. The left panels show epifluorescence microscopy images of cells (ATCC) in suspension after incubation with anti-CD20 antibody-labelled GB1–biosilica (n=3). The right panels show higher-magnification images from the same area. Green: biosilica (GFP-labelled), red: Cell Tracker Orange-stained cells, blue: Cell Tracker Blue-stained cells. (a) B cells (Burkitt’s lymphoma HR1K cells) and (b) T cells (Jurkat cells). (c) Mixture (1:1) of B cells (red) and T cells (blue). White arrows point to biosilica frustules attached to B cells and the white arrowheads point to biosilica frustules in the vicinity of but not attached to T cells. Scale bars, 20 μm (a,b) and 50 μm (c). Figure 5: Interaction of anti-CD20 antibody-labelled GB1–biosilica with B and T cells in suspension. The left panels show epifluorescence microscopy images of cells (ATCC) in suspension after incubation with anti-CD20 antibody-labelled GB1–biosilica ( n =3). The right panels show higher-magnification images from the same area. Green: biosilica (GFP-labelled), red: Cell Tracker Orange-stained cells, blue: Cell Tracker Blue-stained cells. ( a ) B cells (Burkitt’s lymphoma HR1K cells) and ( b ) T cells (Jurkat cells). ( c ) Mixture (1:1) of B cells (red) and T cells (blue). White arrows point to biosilica frustules attached to B cells and the white arrowheads point to biosilica frustules in the vicinity of but not attached to T cells. Scale bars, 20 μm ( a , b ) and 50 μm ( c ). Full size image We also examined the feasibility of applying these functional antibody-bound GB1–biosilica frustules to adherent tumour cells. GB1–biosilica frustules were functionalized with antibody specific for the p75 neurotrophin receptor (p75NTR) and then were incubated with SH-SY5Y neuroblastoma cells ( Fig. 6a ), which express this receptor, and with BSR cells, clone of immortalized baby hamster kidney fibroblasts, as a negative control ( Fig. 6b ). Fluorescence microscopy analysis revealed that anti-p75NTR-labelled GB1–biosilica frustules readily attached to neuroblastoma cells but not to BSR fibroblasts ( Fig. 6a,b ). This binding was also evident from SEM images ( Fig. 6c ). Therefore, it is possible to target adherent tumour cells with antibody-bound GB1–biosilica. 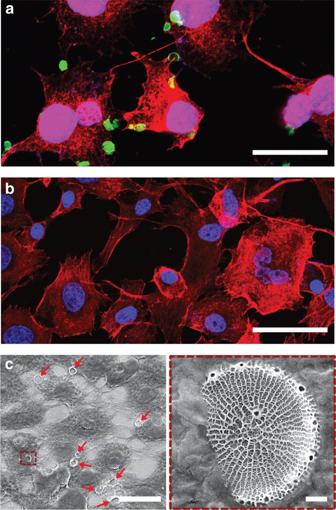Figure 6: Interaction of anti-p75NTR–GB1–biosilica frustules with adherent cells. (a) Confocal fluorescence microscopy image of SH-SY5Y neuroblastoma cells and (b) BSR fibroblast cells (n=3). Red: actin (phalloidin staining, green: biosilica (GFP-labelled), blue: nucleus (Hoechst 33342 staining). (c) The left panel shows an SEM micrograph of SH-SY5Y neuroblastoma cells. Red arrows point to frustules attached to SH-SY5Y neuroblastoma cells. The right panel shows a higher-magnification image of the rectangle framed area inc, which contains a diatom frustule fragment attached to the surface of a cell. Scale bars, 50 μm (a,b), 20 μm (c) and 1 μm (zoom-in area inc). Figure 6: Interaction of anti-p75NTR–GB1–biosilica frustules with adherent cells. ( a ) Confocal fluorescence microscopy image of SH-SY5Y neuroblastoma cells and ( b ) BSR fibroblast cells ( n =3). Red: actin (phalloidin staining, green: biosilica (GFP-labelled), blue: nucleus (Hoechst 33342 staining). ( c ) The left panel shows an SEM micrograph of SH-SY5Y neuroblastoma cells. Red arrows point to frustules attached to SH-SY5Y neuroblastoma cells. The right panel shows a higher-magnification image of the rectangle framed area in c , which contains a diatom frustule fragment attached to the surface of a cell. Scale bars, 50 μm ( a , b ), 20 μm ( c ) and 1 μm (zoom-in area in c ). Full size image Targeted drug delivery to cancer cells in vitro The next step was to load chemotherapeutic drugs onto the GB1–biosilica. Simultaneously loading antibody molecules and chemotherapeutic drugs, which generally are poorly water soluble, is not trivial, as the organic solvents required to dissolve the drug molecules denature the antibody molecules. To circumvent this problem, we used a two-step strategy [20] , [21] . In the first step, a hydrophobic anticancer drug was incorporated into cationic lipid-based colloids (liposomes or micelles). In the second step, the positively charged drug-loaded colloids were adsorbed via electrostatic interactions onto the antibody-labelled biosilica frustules, which have negatively charged surfaces. Camptothecin (CPT; partition coefficient, log P =1.7) and its more potent derivative 7-ethyl-10-hydroxy-CPT (SN38; log P =2.7) were selected as model compounds for poorly water-soluble chemotherapy drugs. CPT-loaded liposomes were prepared with the cationic lipid 1,2-dioleoyl-3-trimethylammonium-propane (DOTAP) [29] and SN38 was encapsulated into cetyltrimethylammonium bromide (CTAB) micelles [30] . The CPT-loaded liposomes and the SN38-loaded micelles had average diameters of ∼ 90 and 115 nm, respectively, and strongly positive ζ-potentials ( Table 1 ). The average ζ-potentials of GB1–biosilica and antibody-labelled GB1–biosilica were approximately −27.6 and −26.0 mV, respectively. This allowed the electrostatic binding of the drug-loaded nanoparticles to the negatively charged antibody-labelled GB1–biosilica and resulted in high drug-loading capacities ( Table 1 ): 0.105 μg CPT and 0.549 μg SN38 per μg of biosilica. The drug-loading efficiency (DL%) was 61.2% for CPT and 85.8% for SN38. Similar DL% values were obtained for biosilica lacking antibody (87.3%). Table 1 Properties of drug-loaded micelles and liposomes. Full size table After drug loading, the antibody-labelled biosilica was dispersed in DMEM medium and the amount of drug released into the medium was determined after incubation at 37 °C for 16 h. About 4% of the biosilica-bound CPT–DOTAP liposomes were released into the medium, resulting in a CPT concentration of 0.16 μg ml −1 , which is more than threefold higher than the minimum toxic dose (0.05 μg ml −1 ) for cancer cells in vitro [31] . Under the same conditions, 1.08 μg ml −1 of SN38 was released from the SN38-loaded, antibody-labelled biosilica into the medium. This is more than 100-fold higher than the minimum toxic dose (0.01 μg ml −1 ) in vitro [32] . These results confirm that the drug-loaded, antibody-labelled GB1–biosilica can release anticancer drugs to concentrations exceeding the minimum toxic dose. We then investigated whether antibody-labelled GB1–biosilica loaded with CPT–DOTAP liposomes or SN38–CTAB micelles can target and kill cancer cells in vitro . Anti-p75NTR–GB1–biosilica was found to be non-toxic towards SH-SY5Y neuroblastoma cells: 92–96% of SH-SY5Y cells and BSR cells remained viable after treatment for 2 days ( Fig. 7 ). Both SH-SY5Y and BSR cells were also highly viable when incubated with GB1–biosilica lacking either the targeting antibody or the liposome- or micelle-encapsulated drugs. By contrast, treatment with anti-p75NTR–GB1–biosilica loaded with CPT–DOTAP liposomes resulted in only 9% of neuroblastoma cells remaining viable after 2 days ( Fig. 7a ), whereas 92% of control fibroblasts were viable ( Fig. 7a ). Similar results were obtained for the anti-p75NTR–GB1–biosilica with adsorbed SN38–CTAB micelles: ∼ 10% of SH-SY5Y cells remained viable after 2 days, whereas 95% of BSR cells were viable ( Fig. 7b ). These results show that drug-loaded, antibody-labelled GB1–biosilica induced cell death, and that this was specific to the neuroblastoma-targeting ability of antibody-labelled GB1–biosilica. 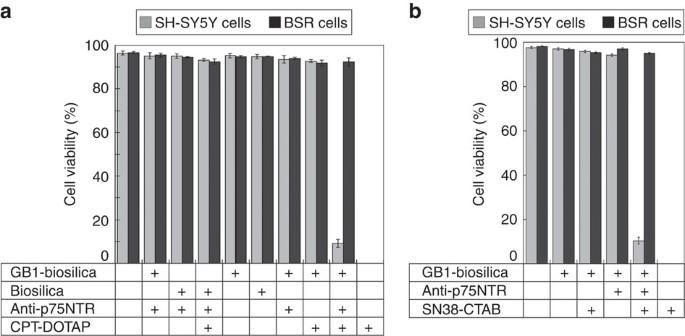Figure 7: Viability of SH-SY5Y neuroblastoma cells targeted by antibody-labelled and drug-loaded biosilica. SH-SY5Y cells (p75NTR positive) and BSR (p75NTR negative) cells were incubated with control samples and with anti-p75NTR–GB1–biosilica that was loaded either with CPT or SN38 (n=3). After 1 h, the medium was replaced to remove unattached biosilica. For each sample, viability analysis was performed in triplicates. (a) Biosilica samples were applied at final concentrations of 20 μg biosilica per ml of cell suspension, corresponding to 2.12 μg ml−1CPT in the case of CPT–DOTAP-loaded biosilica. The concentration of free CPT-loaded liposomes (toxic control) was 1.70 μg CPT per ml. (b) Biosilica samples were applied at final concentrations of 20 μg per ml of cell suspension, corresponding to 10.98 μg ml−1SN38 (loaded in CTAB micelles). For the toxic control, SN38-CTAB micelles were added at a final concentration of 9.30 μg ml−1. For the toxic controls, the medium replacement step after 1 h of incubation was omitted. Error bars represent s.e.m. Figure 7: Viability of SH-SY5Y neuroblastoma cells targeted by antibody-labelled and drug-loaded biosilica. SH-SY5Y cells (p75NTR positive) and BSR (p75NTR negative) cells were incubated with control samples and with anti-p75NTR–GB1–biosilica that was loaded either with CPT or SN38 ( n =3). After 1 h, the medium was replaced to remove unattached biosilica. For each sample, viability analysis was performed in triplicates. ( a ) Biosilica samples were applied at final concentrations of 20 μg biosilica per ml of cell suspension, corresponding to 2.12 μg ml −1 CPT in the case of CPT–DOTAP-loaded biosilica. The concentration of free CPT-loaded liposomes (toxic control) was 1.70 μg CPT per ml. ( b ) Biosilica samples were applied at final concentrations of 20 μg per ml of cell suspension, corresponding to 10.98 μg ml −1 SN38 (loaded in CTAB micelles). For the toxic control, SN38-CTAB micelles were added at a final concentration of 9.30 μg ml −1 . For the toxic controls, the medium replacement step after 1 h of incubation was omitted. Error bars represent s.e.m. Full size image Targeted drug delivery in an in vivo subcutaneous tumour model To extend our findings, we investigated whether drug-loaded, antibody-labelled GB1–biosilica was effective at inhibiting tumour growth in vivo . SH-SY5Y neuroblastoma xenografts were established in the flanks of BALB/c nude mice. In this experiment nude mice were used, because they do not reject tumour cells. Once the tumours reached 150 mm 3 on day 12, mice were randomized into groups ( n =4) and treated with a single intraperitoneal injection of GB1–biosilica (10.78 mg kg −1 ), anti-p75NTR–GB1–biosilica (10.78 mg kg −1 ), anti-p75NTR–GB1–biosilica loaded with SN38–CTAB micelles (10.78 mg kg −1 , equivalent to a dose of 2.25 mg kg −1 SN38) and SN38–CTAB micelles alone (8.90 mg kg −1 , equivalent to a dose of 3.38 mg kg −1 SN38). Tumour growth was then monitored for 15 days. Tumour volumes on day 17 (5 days post treatment) were significantly lower in the anti-p75NTR–GB1–biosilica–SN38–CTAB group than in the GB1–biosilica group ( P =0.002, Student’s t -test), the SN38–CTAB micelle group ( P =0.004, Student’s t -test) or the anti-p75NTR–GB1–biosilica group ( P =0.001, Student’s t -test), by 53%, 47% and 44%, respectively, ( Fig. 8a ). There was a significant interaction between the effects of anti-p75NTR–GB1–biosilica–SN38–CTAB and all other treatment groups on tumour volume (two-way analysis of variance, F (3,21) =7.261 P =0.002). More importantly, tumour regression was observed only in the anti-p75NTR–GB1–biosilica–SN38–CTAB group ( Fig. 8b ). These data demonstrate that antibody-labelled GB1–biosilica enables targeted delivery of hydrophobic chemotherapy drugs in vivo , to achieve a significant reduction in tumour growth in a single dose. 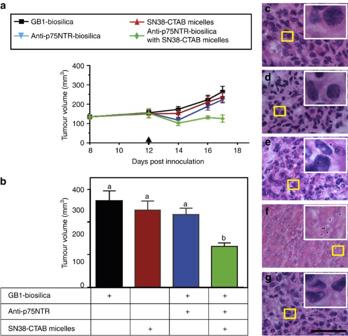Figure 8: Antibody-labelled diatom biosilica loaded with SN38 reduces neuroblastoma SH-SY5Y tumour growth and histochemical analysis of SH-SY5Y xenografts. (a) Average tumour volumes measured over 17 days in immunodeficient Balb/c nude mice that were implanted with SH-SY5Y neuroblastoma cells and treated with single dose of different diatom biosilica-based materials: GB1–biosilica (n=4, black squares), anti-p75NTR–GB1–biosilica (n=4, blue triangles), anti-p75NTR–GB1–biosilica–SN38 (n=4, green diamonds) and SN38–CTAB micelles alone (n=4, red triangles). (b) Comparison of average tumour volumes after 17 days of treatment with anti-p75NTR–GB1–SN38 (green), GB1–biosilica (black), SN38–CTAB micelles (red) and anti-p75NTR–GB1–biosilica (blue). Arrow indicates day on which the intraperitoneal injection was administered. All data are presented as mean±s.e.m. Statistics by analysis of variance (a) and Student’st-test (b). Letters that are not shared are significantly different (a:P=0.002;b:P=0.004). Frozen sections from individual tumours (28 days after tumour cell inoculation) from the following treatment groups (n=4) were stained with H&E. (c) Untreated tumour control. Tumour treated with (d) GB1–biosilica, (e) anti-p75NTR–GB1-labelled biosilica, (f) anti-p75NTR–GB1–biosilica–SN38–CTAB micelles and (g) SN38–CTAB micelles. Treatments via intraperitoneal injection occurred 12 days after tumour cell inoculation. Images are representative of tissue sections selected from four independent experiments (three images for each sample). Insets: dark spots show the diatom biosilica. Scale bar, 50 μm. Figure 8: Antibody-labelled diatom biosilica loaded with SN38 reduces neuroblastoma SH-SY5Y tumour growth and histochemical analysis of SH-SY5Y xenografts. ( a ) Average tumour volumes measured over 17 days in immunodeficient Balb/c nude mice that were implanted with SH-SY5Y neuroblastoma cells and treated with single dose of different diatom biosilica-based materials: GB1–biosilica ( n =4, black squares), anti-p75NTR–GB1–biosilica ( n =4, blue triangles), anti-p75NTR–GB1–biosilica–SN38 ( n =4, green diamonds) and SN38–CTAB micelles alone ( n =4, red triangles). ( b ) Comparison of average tumour volumes after 17 days of treatment with anti-p75NTR–GB1–SN38 (green), GB1–biosilica (black), SN38–CTAB micelles (red) and anti-p75NTR–GB1–biosilica (blue). Arrow indicates day on which the intraperitoneal injection was administered. All data are presented as mean±s.e.m. Statistics by analysis of variance ( a ) and Student’s t -test ( b ). Letters that are not shared are significantly different ( a : P =0.002; b : P =0.004). Frozen sections from individual tumours (28 days after tumour cell inoculation) from the following treatment groups ( n =4) were stained with H&E. ( c ) Untreated tumour control. Tumour treated with ( d ) GB1–biosilica, ( e ) anti-p75NTR–GB1-labelled biosilica, ( f ) anti-p75NTR–GB1–biosilica–SN38–CTAB micelles and ( g ) SN38–CTAB micelles. Treatments via intraperitoneal injection occurred 12 days after tumour cell inoculation. Images are representative of tissue sections selected from four independent experiments (three images for each sample). Insets: dark spots show the diatom biosilica. Scale bar, 50 μm. Full size image The SH-SY5Y tumours were harvested from mice and then sectioned and stained with haematoxylin and eosin (H&E) to observe histopathological changes ( Fig. 8c–g ). Xenografts treated with GB1–biosilica ( Fig. 8d ) or anti-p75NTR–GB1–biosilica ( Fig. 8e ) showed no phenotypical changes in tumour cells compared with the untreated SH-SY5Y tumour ( Fig. 8c ). By contrast, in the group treated with SN38–CTAB micelle-loaded anti-p75NTR–GB1–biosilica, the tumour cells showed vacuolization of their cytoplasm and degeneration of their nuclei ( Fig. 8f ). Biosilica was observed exclusively in tumour tissue from mice treated with anti-p75NTR–GB1–biosilica and anti-p75NTR–GB1–biosilica–SN38–CTAB. The presence of biosilica in the tumour tissue was confirmed by SEM and EDAX ( Supplementary Fig. 4 ). Taken together, these results demonstrate that anti-p75NTR–GB1–biosilica–SN38–CTAB and anti-p75NTR–GB1–biosilica accumulated and degraded in tumour site. Biodistribution of and tissue damage by diatom biosilica To assess the possible side effects of administering biosilica, we conducted in vivo biodistribution studies and assessed whether tissue damage was caused by GB1–biosilica and anti-p75NTR–GB1–biosilica. After a single intravenous injection into nude mice, animals were observed daily for 8 days and the major organs were then collected. In this experiment, nude mice were used for consistency with the subcutaneous tumour model experiment. During observation, none of the mice exhibited any observable symptoms of acute tissue damage. Optical microscopy studies on tissue sections (8 μm) did not reveal any noticeable abnormality in the major organs, the brain, heart, kidney, liver and lung, or the tail. Degraded diatom biosilica was observed in liver and kidney sections but not in the lung ( Fig. 9 , dark spots) and this was confirmed by SEM and EDAX ( Supplementary Fig. 5 ). 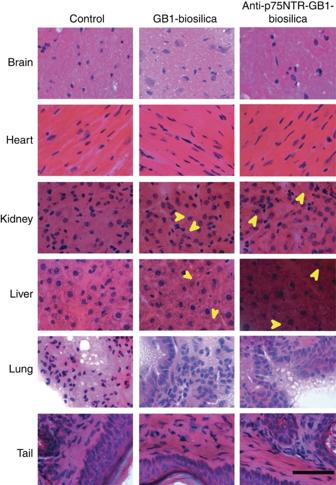Figure 9:In-vivobiodistribution and tissue damage studies of anti-p75NTR–GB1–biosilica. H&E-stained light microscopy images of major organs (the brain, heart, kidney, liver, lung and tail) for Balb/c nude mice treated with GB1–biosilica (n=2) and anti-p75NTR–GB1–biosilica (n=2) for 8 days. The tissues appear normal, some biosilica fragments are evident in the kidney and liver samples of mice treated with GB1–biosilica and anti-p75NTR–GB1–biosilica. Yellow arrows point to biosilica in tissue sections. Images are representative of tissue sections selected from two independent experiments (three images for each sample). Scale bar, 50 μm. Figure 9: In-vivo biodistribution and tissue damage studies of anti-p75NTR–GB1–biosilica. H&E-stained light microscopy images of major organs (the brain, heart, kidney, liver, lung and tail) for Balb/c nude mice treated with GB1–biosilica ( n =2) and anti-p75NTR–GB1–biosilica ( n =2) for 8 days. The tissues appear normal, some biosilica fragments are evident in the kidney and liver samples of mice treated with GB1–biosilica and anti-p75NTR–GB1–biosilica. Yellow arrows point to biosilica in tissue sections. Images are representative of tissue sections selected from two independent experiments (three images for each sample). Scale bar, 50 μm. Full size image Overall, the data presented here show that the proposed strategy for simultaneously labelling diatom biosilica with antibodies and loading with chemotherapeutic drugs is feasible. Moreover, this functionalized and drug-loaded biosilica specifically targets and kills tumour cells. Overall, our approach shares some similarities with the polyelectrolyte multilayer patches developed by Rubner and colleagues [33] . These patches also attach to cells and release drug cargo [33] , but they do not incorporate selective targeting molecules, have limited drug-loading capacity and require an expensive photolithographic approach for patch fabrication. Before drug delivery systems can effectively be used as treatments, their efficiency and cancer specificity must be improved. Much attention has been paid to developing drug carriers that are natural, biocompatible and biodegradable, and that can both bind to biomolecules and recognize unique cell-specific markers. Functionalized biosilica frustules meet all of these criteria. A key step in our process was the in vivo incorporation of a GB1-bearing fusion protein into diatom biosilica through genetic engineering. The GB1 fusion protein was stably attached to the biosilica and accessible for IgG binding, as determined by labelling the genetically modified diatoms with fluorochrome-conjugated antibody. Furthermore, we were able to assess the antibody site density on the diatom biosilica surface by using gold-nanoparticle-labelled IgG in combination with SEM. To investigate the specificity of cell targeting, several antibodies were bound to the biosilica drug carrier. We used anti-CD20 antibody, because it targets a highly expressed cell surface marker of B cells, CD20 (ref. 26 ). The cell-targeting ability of GB1–biosilica frustules labelled with anti-CD20 antibody was confirmed by their binding to immobilized Burkitt’s lymphoma B cells in microarray experiments but not Jurkat T cells, which lack the CD20 marker, indicating that the adhesion of the functionalized biosilica to the cells resulted from specific binding to cell surface proteins. This was also confirmed in mixed cell populations. Furthermore, antibody-mediated targeting of tumour cells was demonstrated by using an antibody that recognizes an antigen on an adherent cancer cell line. Attachment of anti-p75NTR-labelled GB1–biosilica frustules to SH-SY5Y neuroblastoma cells [34] , which express p75NTR, but not to control fibroblasts demonstrated the selective cell targeting of the frustules in an adherent cell system. Therefore, functionalized diatom biosilica can selectively target both adherent and suspension tumour cells. After confirming the selectivity of antibody-labelled GB1–biosilica frustules for specific cell types, we loaded these diatoms with chemotherapeutic drugs and applied them as a targeted drug delivery system. Both of the drugs used, CPT and SN38, are potent chemotherapeutic agents. They exert their activity by binding to the complex formed by DNA topoisomerase I and DNA. This results in a stable ternary complex, thus preventing DNA re-ligation and causing DNA damage and cell death [35] . Despite being potent chemotherapeutics, the poor solubility of CPT and SN38 in most pharmaceutically accepted solvents limits their clinical application. The challenging task of loading hydrophobic chemotherapy drugs onto the antibody-labelled biosilica was solved by electrostatic adsorption of drug-loaded, positively charged liposomes and micelles for later deployment. Up to 85.8% DL% was achieved, which is higher than has been reported for other nanoparticle systems [36] . For both liposomal and micellar nanocarriers adsorbed to diatom biosilica, release studies showed that more than the required effective drug dose was released into the culture medium, indicating the potential to kill targeted cells. Selective killing of neuroblastoma cells was subsequently shown using antibody-labelled drug-loaded biosilica, whereas control cells remained highly viable in vitro . When anti-p75NTR–GB1–biosilica loaded with liposomes or micelles encapsulating drug was incubated with SH-SY5Y cells, cell viability decreased to 9–10%, demonstrating the successful delivery of CPT and SN38 to neuroblastoma cells by our nanoparticle delivery system. Moreover, anti-p75NTR-labelled GB1–biosilica loaded with SN38–CTAB micelles reduced tumour growth in SH-SY5Y neuroblastoma tumour-bearing BALB/c nude mice 5 days post intraperitoneal administration. This significant therapeutic effect was specific, because there was clear evidence of biosilica within the tumour tissue sections of mice that had been treated with the anti-p75NTR antibody-labelled biosilica but none in mice treated with the non-targeted biosilica. Therefore, our system enables targeted delivery of a hydrophobic chemotherapy drug in vivo and results in a significant reduction in tumour growth with a single dose, in contrast to chemotherapy drug alone or antibody-labelled biosilica without drug. Biodistribution experiments showed that both functionalized and non-functionalized GB1–biosilica was observed in the liver and kidney but not in other vital organs of mice. The accumulation of both targeted and non-targeted nanoparticles in the liver and kidney has also been reported in previous studies [37] , [38] . The liver accumulation of silica is expected as a result of particle uptake by macrophages in the reticuloendothelial system [39] . In conclusion, we established the use of diatom biosilica, a natural mesoporous silica material, for use in targeted drug delivery. Our work therefore paves the way for a novel drug delivery system using a biotechnologically tailored, renewable material. Cultivation of T. pseudonana T. pseudonana (Hustedt) Hasle et Heimdal clone CCMP1335 was grown in an enriched artificial seawater medium according to the North East Pacific Culture Collection protocol (Canadian Centre for the Culture of Microorganisms, ESAWRecipe) at 18 °C under constant light at 5,000–10,000 lux [22] . The composition of the enriched artificial seawater medium per 1 l (adjusted to pH 8.2 with NaOH) was: 20.8 g NaCl, 9.6 g MgCl 2 ·6H 2 O, 3.5 g Na 2 SO 4 , 9 mM CaCl 2 , 8 mM KCl, 47 mg NaNO 3 , 21 mg SrCl 2 ·6H 2 O, 30 mg Na 2 SiO 3 ·9H 2 O, 6 mg Na 2 EDTA·2H 2 O, 33 μg ZnCl 2 , 20 μg CoCl 2 ·6H 2 O, 130 μg Na 2 MoO 4 ·2H 2 O, 500 μg MnCl 2 ·4H 2 O, 25 mg H 3 BO 3 , 17 μg Na 2 SeO 3 ·5H 2 O, 2 mg FeCl 3 ·6H 2 O, 3 mg KF, 85 mg KBr, 6 mg Na 2 -glycerophosphate·H 2 O, 100 mg NaHCO 3 , 200 μg thiamin·HCl, 4 μg vitamin B12 and 2 μg biotin. Cloning of the T8–GB1–GFP fusion gene The gene encoding enhanced GFP, egfp , was PCR amplified from plasmid pTpNR/ egfp [17] using the oligonucleotides 5′-GATC CTG CAG ATG GTG AGC AAG GGC GAG GAG-3′ and 5′-GAAT GCG GCC GC T ACG TA G AAT TC T CCA CCC TTG TAC AGC TCG TCC ATG CC-3′ (PstI site underlined, NotI site in italics and EcoRI site in bold) and then ligated into the PstI and NotI sites of vector pTpNR/T8–PstI egfp NotI, resulting in the plasmid pTpNR/T8– egfp EcoRI–NotI. The unique EcoRI site (bold) and NotI site (italics) at the 3′-end of egfp allowed for the in-frame insertion of genes behind the GFP. A portion of the streptococcal protein G-coding sequence (5′-KTDT YKLILNGKTLKGETTTEA VDAATAEKVFKQYANDNGVDGEWTYDDATKTFTVTE KPE-3′) that includes the IgG-binding domain B1 (underlined) pgb1 (ref. 40 )was PCR amplified from pUC57/ pgb1 (synthesized by Genescript) using the oligonucleotides 5′- GAA TTC AAG ACT GAC ACT TAC AAA TTA AT-3′ and 5′- GCG GCC GC T TAT TCT GGT TTT TCA GTA ACT GTA A-3′(EcoRI site in bold and NotI site in italics) and then ligated into the EcoRI and NotI sites of vector pTpNR/T8– egfp EcoRI–NotI, resulting in the final plasmid pTpNR/T8– egfp – pgb1 . All PCR products were verified by DNA sequencing. The plasmid constructs were introduced into T. pseudonana cells by microparticle bombardment using an established method [25] , [40] . Transformant clones were selected on agar plates containing the antibiotic nourseothricin. Nourseothricin-resistant clones were picked from the agar plates and grown in liquid medium containing the antibiotic. Cells were screened for the presence of the GFP fusion protein using a Zeiss Axioplan 200 epifluorescence microscope equipped with a Piston GFP bandpass filter set (Ex: HQ470/ × 40, Dichroic Q495LP, Em: HQ515/30 M; Chroma Technology Corp.). Isolation of diatom biosilica T. pseudonana cell transformants were resuspended in PBS buffer (20 mM sodium phosphate pH 7.5, 150 mM NaCl, 1 × protease inhibitor cocktail) and then lysed by vortexing (three times, 30 s) with glass beads (diameter, 0.25–0.30 mm). The lysate was centrifuged (5 min, 10,000 g , 4 °C) and the pellet was washed three times with PBS buffer. The pellet was then extracted five times by centrifugation–resuspension with 1 vol% Igepal-CA630 (in PBS buffer) at 4 °C for 5 min each. The remaining biosilica was washed five times with PBS buffer by centrifugation (5 min. 10,000 g , 4 °C)–resuspension and then resuspended in PBS buffer containing a protease inhibitor cocktail. IgG binding to diatom biosilica T8–GFP–GB1–biosilica or T8–GFP–biosilica (each ∼ 1 mg wet weight) were incubated with 5 μg of anti-rabbit IgG-HRP (Sigma-Aldrich) in 1 ml PBS buffer overnight with rotation at 4 °C. The biosilica was then washed three times with PBS buffer by centrifugation (5 min, 10,000 g , 4 °C)–resuspension and then twice with potassium phosphate buffer (78 mM, pH 6.0). The activity of anti-rabbit IgG–HRP-bound biosilica was quantified by incubation in 200 μl assay buffer (3.9 mM H 2 O 2 , 78 mM potassium phosphate, pH 6.0, 17 μM n-octadecyltrimethoxysilane) at room temperature for 20 min. Subsequently, the biosilica was pelleted by centrifugation (5 min, 16,000 g ) and the absorbance of the supernatant was measured at 410 nm. In a separate experiment, T8–GFP–GB1–biosilica and T8–GFP–biosilica (control) (200 μg ml −1 ) were incubated with 1 mg ml −1 DyLight 549-conjugated mouse antihuman IgG (Abcam) for 16 h at 4 °C. The biosilica frustules were then washed with sterile PBS, to remove excessive and unattached antibodies by centrifugation at 1,000 g for 3 min at 8 °C. The biosilica was then examined with an inverted fluorescence microscope (Nikon Eclipse Ti-S). T8–GFP–GB1–biosilica or T8–GFP–biosilica were dispersed at 200 μg ml −1 concentration in anti-CD20 antibody solution (1 mg ml −1 ) and incubated for 16 h at 4 °C. Anti-CD20 antibody (Roche) was kindly provided by Dr Peter Macardle (Department of Immunology at Flinders Medical Centre, Australia). Unbound anti-CD20 antibodies were removed by centrifuging diatom preparations at 1,000 g for 3 min at 8 °C, followed by three subsequent 5 min washes in PBS at room temperature and finally dispersed in PBS. The same experiment was performed with the anti-p75NTR mouse monoclonal antibody (MLR2) [41] . Anti-p75NTR antibodies were kindly provided by Mary-Louise Rogers (Department of Human Physiology, Centre for Neuroscience, Flinders University, South Australia, Australia). Determination of IgG density bound to diatom biosilica T8–GFP–GB1–biosilica and T8–GFP–biosilica (control; 200 μg ml −1 ) were incubated for 16 h at 4 °C with 1.7 × 10 13 particles per ml of anti-rat IgG conjugated to a 10-nm gold nanoparticle (Sigma). The biosilica was then washed with sterile PBS, to remove unattached antibodies by centrifugation at 1,000 g for 3 min at 8 °C. The biosilica was then examined for gold nanoparticles by SEM. Biosilica was deposited on a carbon tape and then imaged using a SEM (FEI Quanta 450-FEG) at 10 keV. The presence of gold was confirmed by EDAX (Apollo X SDD). The gold particle density was obtained by manually counting the particles in the SEM micrographs. Preparation of CPT-loaded DOTAP liposomes Powdered DOTAP (Avanti Polar Lipids) was dissolved in chloroform/methanol (2:1 vol/vol) to make a 25 mg ml −1 stock solution. CPT (Sigma-Aldrich) was dissolved in dimethylsulphoxide, to produce a 4 mg ml −1 stock solution. CPT and DOTAP stock solutions were combined to make 1:1 mixture (1 ml) and the solvents were then evaporated under a constant stream of nitrogen gas for ∼ 60 min. The residue was dissolved in PBS buffer (Na 2 HPO 4 , NaCl, KH 2 PO 4 , KCI, pH 7.4) to final concentrations of 12.5 mg ml −1 DOTAP and 2 mg ml −1 CPT. The solution was placed in an ultrasonic bath for 30 min and subjected to intermittent vortex mixing (it is noteworthy that the solution was completely transparent at this stage). Following sonication, 1 ml of the lipid–CPT mixture was extruded 21 times through a 50-nm porous polycarbonate membrane (Avanti Polar Lipids) using a handheld extruder (ATA Scientific). The resulting solution was used for loading onto the diatom biosilica. Preparation of SN38-loaded cationic micelles The solution of CTAB (Sigma-Aldrich) at 2 mg ml −1 was prepared, which is above the critical micelle concentration at the temperature studied in this work. SN38 (purity of 99%, Flourish Pharma Limited, Hong Kong, China) was dissolved at 1 mg ml −1 in 0.1 mM NaOH (it is noteworthy that at pH 10, SN38 is present in the carboxylate form). The drug was incorporated into CTAB micelles by vigorously stirring a 1:2 (w/w) mixture of SN38 and CTAB for 20 min. The pH of the mixture was then adjusted to pH 2 by the addition of HCl (0.1 M), which converted SN38 to the lactone form. The hydrophobic lactone was allowed to incorporate into the hydrophobic core of CTAB micelles overnight under magnetic stirring, the pH of the mixture was then adjusted to neutral condition (7.2–7.4) with 0.1 M NaOH and final CTAB micelles were obtained following the precipitation of the unloaded drug by centrifugation at 1,800 g for 10 min. CTAB micelles were resuspended in PBS to a final concentration of 380 μg SN38 per ml. Liposome and micelle characterization Particle sizes and ζ-potentials of the drug-loaded liposomes and micelles were characterized by dynamic light scattering and phase analysis light scattering using the Zetasizer Nano (Malvern), respectively. Milli Q water (refractive index=1.33) was used as the dispersant; the particle refractive index was pre-set as 1.336 for CTAB micelles and 1.345 for liposomes. Measurements were carried out at 25 °C. Size distributions are expressed as the z -average diameter together with the polydispersity index. ζ-Potentials are presented as the mean of more than ten measurements. Drug-loaded liposome and micelle loading on diatom biosilica CPT–DOTAP liposomes (34.6 μg CPT per ml) were added to a suspension of 200 μg ml −1 anti-p75NTR–GB1–biosilica in PBS. The mixture was then incubated at 4 °C for 16 h. Following incubation, the biosilica was pelleted by centrifugation (1,000 g , 5 min, 8 °C) and the supernatant was transferred into another microfuge tube. The biosilica in the pellet phase was subsequently washed with PBS by adding PBS (0.5 ml) to the pellet, resuspended by gentle pipetting and centrifugation (1,000 g , 5 min, 8 °C). The final pellet was considered the CPT–DOTAP liposome-loaded biosilica. Supernatants formed in both centrifugation processes were collected; they were diluted properly with HPLC mobile phase and analysed for the drug content by the HPLC method described below. The amount of CPT attached to the biosilica was calculated by subtracting the amount of CPT in the supernatants from the initial amount of CPT added. The amount of CPT attached to the biosilica was divided by the initial amount and was calculated as the DL%. To determine the rate of release of CPT into DMEM following 16 h incubation of CPT–DOTAP liposomes-loaded biosilica (2.12 μg CPT per ml) (37 °C, 5% CO 2 ), an aliquot of 0.5 ml sample was collected and centrifuged (1,000 g , 5 min, 8 °C). The supernatant was collected, diluted to the range within 0.05–50 μg ml −1 and analysed for CPT content by HPLC. Anti-p75NTR–GB1–biosilica was loaded with SN38–CTAB micelles following the same method as described above for CPT–DOTAP liposomes. Specifically, 100 μl of a biosilica suspension (200 μg ml −1 ) was incubated with 200 μl SN38–CTAB micelles (380 μg SN38 per ml) for 16 h at 4 °C. The biosilica was pelleted by centrifugation at 1,000 g for 5 min at 8 °C and the supernatant was transferred into another microfuge tube. The biosilica in the pellet phase was subsequently washed with PBS by adding PBS (0.5 ml) to the pellet, resuspended by gentle pipetting and centrifugation (1,000 g , 5 min, 8 °C). The final pellet was considered the SN38–CTAB micelle-loaded biosilica. Supernatants formed in both centrifugation processes were collected; they were diluted to the range within 0.05–50 μg ml −1 with HPLC mobile phase and analysed for the drug content by HPLC method described below. The amount of SN38 attached to the biosilica was calculated by subtracting the amount of SN38 in the supernatants from the initial amount of SN38 added. To determine the rate of release of SN38 into cell culture medium following 16 h incubation of SN38–CTAB micelle-loaded biosilica (10.98 μg CPT per ml) (37 °C, 5% CO 2 ), an aliquot of 0.5 ml sample was collected, extracted with dimethylsulphoxide (1.5 ml), sonicated for 5 min and centrifuged (1,000 g , 5 min, 8 °C). The supernatant was collected, diluted to the range within 0.05–50 μg ml −1 and analysed for SN38 content by HPLC. HPLC analysis CPT and SN38 was assayed using a HPLC system (Shimadzu Corporation) consisting of a series of LC-20ADXR pumps, SIL-20ACXR auto sampler, CTO-20AC column oven and SPD20A variable ultraviolet detector set at 380 nm, and a LiChrospher C18 analytical column (RP-18, 5 μm, 4.6 mm ID × 250 mm). The mobile phase was a mixture of acetonitrile and 10 mM phosphoric acid (5:5 v/v, pH 3.0 adjusted by addition of 1 M NaOH), eluted at a flow rate of 1.2 ml min −1 . The limit of detection and the limit of quantification of this analytical method were 8 and 24 ng ml −1 , respectively for SN38, and 5 and 15 ng ml −1 , respectively for CPT. The intra- and inter-day assay precision was assessed by coefficient of variance (<3% and <5%, respectively) and the accuracy was assessed as percentage bias (<5%). Linear calibration curves ( r 2 ≥0.99) were plotted for chromatographic peak areas against drug concentrations over the range of 0.05–50 μg ml −1 , without the addition of an internal standard due to high specificity and reproducibility of the assay. All analytes were diluted suitably to establish a final concentration in the range for HPLC quantification. Antibody microarray printing Glass microscopy slides were cleaned by rinsing in 70% ethanol and H 2 O, followed by treatment with Piranha solution (40% H 2 SO 4 and 60% H 2 O 2 ) at room temperature for 60 min. The slides were then extensively washed with H 2 O, dried in a stream of air and silanized immediately as described in the following. The samples were dip-coated into a 10% solution of the epoxy silane (3-glycidyloxypropyl) trimethoxysilane (Sigma-Aldrich) in dry toluene at room temperature for 30 min. The slides were then washed extensively with dry toluene, to remove excessive epoxy silane (3-glycidyloxypropyl) trimethoxysilane, and were dried in a stream of dry nitrogen. The modified substrates were then used for antibody printing experiments within 1 h. Anti-CD45 antibody (BD Bioscience; 200 μg ml −1 in sterile Dulbecco’s PBS) was printed on freshly prepared epoxy-silane-coated slides at 65% humidity and 18 °C using a XactII Microarray printer (Labnext) with 350 μm diameter hollow pins (Labnext) [27] , [42] . After printing, arrays were stored at 4 °C for 16 h. To impede nonspecific protein adsorption and cell attachment, the printed slides were incubated in 5% BSA (Sigma-Aldrich) in sterile PBS at pH 7 at 37 °C for 16 h. The arrayed slides were washed with sterile PBS (Sigma-Aldrich). Lymphocyte cell culture experiments The cell lines P3J.HR1K (American Type Culture Collection, ATCC, acute B-cell leukemia) and Jurkat (Clone E6-1, ATCC, acute T-cell leukaemia) cells were maintained in RPMI 1640 medium (Sigma-Aldrich) supplemented with 10% fetal bovine serum (FBS), 100 U ml −1 penicillin and 100 μg ml −1 streptomycin (Invitrogen). Cells were tested for mycoplasma contamination on the day of each experiment and only mycoplasma-free cultures were used. P3J.HR1K and Jurkat cells were stained separately with 10 μM Cell Tracker Orange CMRA (Invitrogen) and 10 μM Cell Tracker Blue CMAC (Invitrogen) for 45 min at 37 °C and 5% CO 2 , respectively. Subsequently, both cell types were mixed at a 1:1 ratio and then incubated with diatoms for 2 h at 37 °C at 5% CO 2 . Antibody microarray slides were pre-treated with 200 U ml −1 penicillin (Invitrogen), 200 μg ml streptomycin (Invitrogen) and 500 ng ml −1 amphotericin B (Invitrogen) in sterile PBS for 4 h. Each slide was placed in a four-well plate (Nunc) and seeded with cells at a density of 1 × 10 5 cells per cm 2 . Cells were incubated on the array for 90 min at 37 °C and 5% CO 2 . Loosely attached cells were then removed by washing with pre-warmed DMEM. The cells were subsequently incubated in fresh DMEM including 10% FBS at 37 °C and 5% CO 2 from 2 to 4 h. Afterwards, T8–GFP–GB1–biosilica or T8–GFP–biosilica were added at 20 μg ml −1 and incubated at 37 °C and 5% CO 2 for 1 h. After three washes with PBS, cells were fixed in 4% paraformaldehyde (Sigma-Aldrich) in PBS for 30 min, then permeabilized with 0.25 % Triton X-100 (Sigma-Aldrich) for 5 min at room temperature. Nuclei of cells were stained with 2 μg ml −1 Hoechst 33342 (Life Technologies) for 15 min at room temperature. Actin filaments were stained with 100 μM phalloidin–tetramethylrhodamine B-isothiocyanate (TRITC) (Sigma-Aldrich) in PBS for 45 min, mounted with Prolong Gold antifade reagent (Invitrogen) and imaged using an inverted fluorescence microscope (Nikon Eclipse Ti-S) equipped with appropriate filters for Hoechst 33342, TRITC-labelled phalloidin and GFP. The percentage of B cells and T cells with attached anti-CD 20 antibody-labelled GB1–biosilica on the microarray spots and in suspension was quantified by manually counting ( n >200 cells). Adherent cell culture and cytotoxicity experiments BSR cells, a clone of baby hamster kidney fibroblast cells (ATCC) and SH-SY5Y human neuroblastoma cells (ATCC) were cultured in DMEM supplemented with 10% FBS, 100 U ml −1 penicillin and 100 μg ml −1 streptomycin (Invitrogen). Cells were tested for mycoplasma contamination on the day of each experiment and only mycoplasma-free cultures were used. SH-SY5Y and BSR cells were placed in wells of a 96-well plate at 10,000 cells per well. After 1 day, SH-SY5Y and BSR cells were incubated with functionalized or non-functionalized biosilica samples for 1 h at 20 μg ml −1 concentration at 37 °C and 5% CO 2 . Following incubation, cells were washed with PBS (three times, 5 min each), to remove unattached biosilica, and incubated in DMEM (10% FBS, 100 U ml −1 penicillin and 100 μg ml −1 streptomycin) in 5% CO 2 at 37 °C for 48 h before cell viability measurements. Confocal fluorescence microscopy To investigate the attachment of biosilica to SH-SY5Y, cells were grown on sterile coverslips at a density of 5 × 10 4 cells per cm 2 . After 1 day of incubation, cells were incubated with antibody-loaded or antibody-free biosilica at 200 μg ml −1 concentration for 1 h at 37 °C and 5% CO 2 . Cells were then washed with PBS, fixed for 10 min in a solution containing 4% paraformaldehyde EM grade (Electron Microscopy Sciences). For confocal fluorescence microscopy, fixed cells were permeabilized with 0.1% Triton X-100 (Sigma-Aldrich) for 5 min at room temperature. Nuclei of cells were stained with 2 μg ml −1 Hoechst 33342 (Life Technologies) for 10 min at room temperature. Actin was stained with 100 μM TRITC-labelled phalloidin (Sigma-Aldrich) for 45 min. Finally, the coverslips were washed in PBS and mounted using fluoro-gel mounting reagent (ProSciTech). Stained cells were imaged using a confocal fluorescence microscope (Nikon A1) equipped with appropriate filters. Images shown are representative of at least three independent experiments and were obtained using identical sensitivity parameters. For SEM, cells on coverslips were fixed, then rinsed twice with Milli Q water and dried in a desiccator under vacuum for 30 min. The dried coverslips were sputter-coated with platinum at a thickness of about 15 nm. SEM was performed using a Quanta 450 (FEI). Samples were observed by collecting secondary electrons at 10 kV beam energy under high vacuum of 6 × 10 −4 Pa. Cell viability experiments To determine the percentage of live and dead cells, lactate dehydrogenase (LDH) released in culture supernatants was measured using an established assay (Abcam LDH-Cytotoxicity Assay Kit II) according to the manufacturer’s instructions. After 48 h incubation with biosilica samples, 100 μl of the cell suspension was centrifuged at 600 g for 10 min and the supernatant was transferred into a 96-well plate. To each well, 100 μl LDH reaction mix was added and after 30 min incubation at room temperature the absorbance at 450 nm was measured. A Live/Dead cell assay was also performed by incubating cells with final concentrations of 15 μg ml −1 fluorescein diacetate (Invitrogen) and 5 μM propidium iodide (Sigma-Aldrich) for 3 min at 37 °C. All experiments were repeated at least three times. In-vivo xenograft studies All animal work was carried out in accordance with The Australian Code of Practice for the Care and Use of Animals for Scientific Purpose 2004 and approved by the Monash Medical Centre Ethics Committee A, approval number 2011/76). Six-week-old female athymic BALB/c nude mice (ARC, Perth, Australia) were housed under specific pathogen-free conditions and provided with food and water ad libitum . Mice were injected subcutaneously in each flank with the neuroblastoma cell line SHSY5Y (10 × 10 6 cells in Matrigel). Tumours were measured twice a week with digital microcalipers and volumes calculated (volume=(width 2 × length)/2). The average tumour volume reached 150 mm 3 on day 12 and the mice were then injected with SN38-CTAB micelles at a concentration of 8.90 mg kg −1 or 142.4 μg per mouse ( n =4), GB1–biosilica at a concentration of 10.78 mg kg −1 or 172.5 μg per mouse ( n =4), anti-p75NTR–GB1–biosilica at a concentration of 10.78 mg kg −1 ( n =4) and anti-p75NTR–GB1–biosilica–SN38 at a concentration of 10.78 mg kg −1 ( n =4) were administered intraperitoneally. Two mice were kept untreated as a control. Tumours were measured daily and once the maximal tumour volume was reached (1,000 mm 3 ), mice were killed. Tumour volumes are represented as mean volume±s.e.m. Tumours were collected and frozen in Tissue-Tek optimum cutting temperature (O.C.T.) freezing compound (Thermo Fisher Scientific, Scoresby, Australia) and stored at −80 °C. Cryosections were prepared with 8 μm thickness. The sections were fixed with cold methanol for 10 min at −20 °C. H&E staining was performed according to a standard procedure. Briefly, the sections on slides were submerged into Lillie-Mayer’s haematoxylin solution (Sigma) for 10 min, then rinsing in tap water for 2 min. Subsequently, the slides were submerged into 2% alcoholic eosin solution (Sigma) for 2 min. Slides were drained well, sections were dehydrated through an ascending alcohol bath series (30, 50, 70, 95 and 100 %, 1 min in each) and cleared in xylene (Sigma) for 2 min. Finally, the slides were allowed to air dry and were mounted in distrene plasticiser xylene mountant for histology (Sigma). Biodistribution studies For biodistribution analysis of tissues, a second set of Balb/c nude mice were injected intravenously into the tail vein with GB1–biosilica ( n =2) or anti-p75NTR–GB1–biosilica ( n =2) at a concentration of 3.23 mg kg −1 or 51.75 μg per mouse. Two untreated nude mice were used as control. After 8 days, various organs (the heart, liver, lungs, kidneys, brain and tail) were harvested and frozen in Tissue-Tek O.C.T. freezing compound and stored at −80 °C. Histology of organs Organs embedded in O.C.T. were cryosectioned. Frozen tissue sections of 8 μm thickness were fixed with cold methanol for 10 min at −20 °C and stained using H&E according to a standard procedure, for visualization of the nucleus and cytoplasm. Evaluation of each sample was performed by a certified haematopathologist using a light microscope (Nikon Eclipse Ci). The sections were then examined for biosilica by SEM. Sections was deposited on a carbon tape and then imaged using a FEI Quanta 450-FEG SEM at 10 keV. The presence of biosilica was confirmed by EDAX on an Apollo X SDD. Statistical analysis Statistical analyses were carried out using analysis of variance and Student’s t -test analysis, and data were considered statistically significant when P <0.05. All tests were performed using Graph Pad Prism for Windows version 6.02. How to cite this article: Delalat, B. et al. Targeted drug delivery using genetically engineered diatom biosilica. Nat. Commun. 6:8791 doi: 10.1038/ncomms9791 (2015).